Mechanism of Ca2+-triggered ESCRT assembly and regulation of cell membrane repair In muscle and other mechanically active tissue, cell membranes are constantly injured, and their repair depends on the injury-induced increase in cytosolic calcium. Here, we show that injury-triggered Ca 2+ increase results in assembly of ESCRT III and accessory proteins at the site of repair. This process is initiated by the calcium-binding protein—apoptosis-linked gene (ALG)-2. ALG-2 facilitates accumulation of ALG-2-interacting protein X (ALIX), ESCRT III and Vps4 complex at the injured cell membrane, which in turn results in cleavage and shedding of the damaged part of the cell membrane. Lack of ALG-2, ALIX or Vps4B each prevents shedding, and repair of the injured cell membrane. These results demonstrate Ca 2+ -dependent accumulation of ESCRT III-Vps4 complex following large focal injury to the cell membrane and identify the role of ALG-2 as the initiator of sequential ESCRT III-Vps4 complex assembly that facilitates scission and repair of the injured cell membrane. Owing to mechanical activity, the myofibre’s cell membrane (sarcolemma) is exposed to constant injury [1] , [2] . In the face of frequent injury, muscle cells depend on efficiently repairing tears in their sarcolemma—this is a Ca 2+ -dependent process [2] , [3] . Cell membrane repair involves use of intracellular compartments, which in case of muscle cells include mitochondria [4] , lysosomes [5] , [6] and caveolae [7] . These compartments perform different functions during repair of the injured cell membrane. Mitochondria accumulate at the site of injury, lysosomes fuse with the injured cell membrane to secrete acid sphingomyelinase, and caveolae internalize pores in the injured cell membrane [4] , [6] , [7] , [8] . Thus intracellular compartments facilitate repair of injured cell membrane by various processes including clotting, patching or removing the damaged portions of the injured cell membrane [4] , [9] , [10] . The process of endocytic removal of plasma membrane wound by pore forming toxins (pores of <100 nm) has been shown to involve exocytosis of lysosomes and endocytosis through caveolae as well as ESCRT-mediated budding of intraluminal vesicles in the late endosome [8] . Shedding (ectocytosis) of small (<100 nm) plasma membrane wounds, facilitated by ESCRTs, has also been shown to aid in repair of such cell membrane wounds [11] , [12] . Unlike pore-forming toxins, exercise and other muscle injuries lead to large (micron scale) wounds in the cell membrane, but the processes leading to their repair is not well elucidated [1] , [13] . Repair of large mechanical injury to muscle involves increased caveolar endocytosis [7] , which is initiated by acid sphingomyelinase (ASMase) released owing to injury-triggered lysosomal exocytosis [14] . We found that muscle cell injury also triggers lysosome exocytosis resulting in ASMase secretion, a defect in which compromises repair of the injured myofibres [6] . In addition to triggering caveolar endocytosis, ASMase also causes shedding of plasma membrane vesicle [15] . However, the role of plasma membrane shedding (ectocytosis) in repair of large cell membrane wound has not been established. Irrespective of the size of the cell membrane wound and the cellular mechanism involved in its repair, a common feature of all of these processes is their dependence on the increase in cytosolic Ca 2+ . Thus, to understand the molecular process involved in repair of muscle cell membrane, we analyzed Ca 2+ -induced changes in muscle cell membrane proteome. This identified that Ca 2+ triggers accumulation of ESCRT complex at the cell membrane. Live imaging of muscle and other cells undergoing repair from large (>1 μm) focal injury confirmed Ca 2+ -triggers translocation of ESCRTs and accessory proteins at the site of repair. Ca 2+ - and injury-triggered ESCRT accumulation is initiated by a calcium-binding protein ALG-2 (apoptosis-linked gene-2) and its interacting protein ALIX (ALG-2 interacting protein X) [16] . Injury-triggered ESCRT assembly culminates in accumulation of Vps4, which aids in cleavage and shedding of the damaged cell membrane. Shedding and repair of injured cell membrane was prevented in cells lacking ALG-2, ALIX or Vps4B. Our findings demonstrate repair of large cell membrane injury as a new role of ESCRT-mediated membrane scission. This adds to the known role of ESCRTs in the formation of intraluminal vesicles [17] , retrovirus budding [18] , [19] , cytokinesis [20] , [21] , [22] and repair of nanometer scale cell membrane wounds due to pore-forming toxins [8] . Similar to the latter [19] , [22] , [23] , we find ESCRT-mediated cell membrane repair makes use of a non-ESCRT protein (ALG-2) to initiate assembly of ESCRT III and Vps4 complexes. These results point to a role of ESCRT complex in repair of large injuries, and identify the mechanism for ESCRT III assembly triggered by large cell membrane injury. Acute increase in Ca 2+ changes cell membrane proteome To quantify Ca 2+ -induced changes in the muscle cell membrane proteome, we carried out mass spectrometry for quantitative proteomics with stable isotope labelling by amino acids in cell culture (SILAC). Using this approach, we previously identified mitochondria as a cellular compartment needed for the repair of injured myofibres [4] . Here we extended this approach to mononucleated muscle cells and analyzed the change in cell membrane proteome of C2C12 myoblasts treated for 5 min with either 0.1% dimethylsulphoxide (DMSO) (control) or with 10 μM Ca 2+ ionophore—ionomycin. To obtain proteins reproducibly altered in response to ionomycin, we carried out six replicate pairs such that in five replicates SILAC-labelled cells were treated with ionomycin and in one replicate they were treated with DMSO. Each pair was then mixed and proteins were resolved by sodium dodecyl sulfate polyacrylamide gel electrophoresis ( Fig. 1a ). This identified 1,556 protein pairs that were detected in two or more replicates ( Supplementary Data 1 ). Averaging the ratio of extracted spectral intensity of each SILAC- labelled and -unlabelled peptide detected for a protein provided ionomycin-induced fold-change for each protein. The log 2 fold change s.d. across the 1,556 proteins was ±0.4. Next, we calculated each protein’s P value independently using one sample t -test to determine the statistical significance of difference in the values obtained for a given sample with respect to the null hypothesis of a change in ratio of 1. Proteins that differed significantly ( P <0.06; one sample t -test versus ratio of 1.0) from an unaltered ratio of 1 (log2=0) were identified. Applying filters of P value <0.06 and log 2 s.d. ±0.2 (ratio cutoff of ≥1.15 or ≤0.87), narrowed the list to top 10% of altered proteins (130 increased and 24 decreased) ( Supplementary Data 2 , Fig. 1b ). Owing to the small fold changes, we attempted to validate Ca 2+ -triggered changes in the cell surface level of proteins reported by mass spectrometry (MS) analysis independently by western blot (WB) analysis. We found that while the magnitude of change varies between MS and WB analyses, each of the dozen proteins assayed by WB analysis exhibited the same trend of Ca 2+ -triggered change at the cell surface level as predicted by MS analysis. Representative proteins that showed ionomycin-induced increase in cell membrane level by MS analysis—Galectin-1 (fold change 1.76±0.01; P value 0.008) and Annexin A1 (fold change 1.27±0.03; P value 0.026) also showed increased level by WB analysis ( Fig. 1c ). Similarly, proteins whose level did not change, for example: Cadherins (fold change 0.94–1.1; P value >0.72) ( Supplementary Data1 ) were found to be unaltered by WB analysis using pan-Cadherin antibody ( Fig. 1c ). 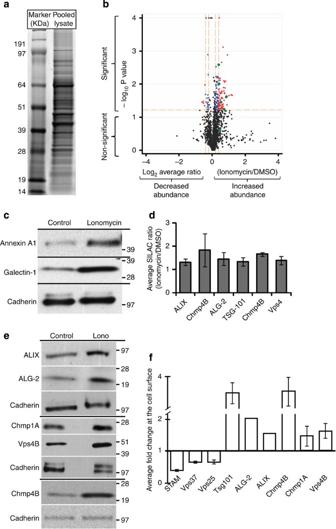Figure 1: Ca2+triggers recruitment of ESCRT III complex at the cell membrane. SILAC labelled and unlabelled C2C12 myoblasts treated for 5 min with Ionomycin (10 μM) or with DMSO (0.1%) were pooled, and the cell membrane proteins were extracted. (a) A representative coomassie-stained 1D SDS-PAGE gel (n=6) used for differential cell membrane proteomic analysis. The gel shows molecular weight marker and the cell membrane protein pool (pooled lysate). The gel lane for pooled lysate was cut into slices and processed for proteomic analysis by mass spectrometry (MS). (b) Scatter (volcano) plot shows the fold change (log2average ratio) and –log10Pvalue (one samplet-test versus ratio of 1.0) for the proteins quantified in at least two of the six independently replicated experiments. Black spots represent protein whose abundance was not altered in response to ionomycin-triggered Ca2+increase or the alteration did not reach the designated statistical significance across replicates. Red symbols represent proteins withP<0.06 (one samplet-test versus ratio of 1.0) and fold change ±0.4 s.d., whereas blue symbols mark proteins withP<0.06 and fold change ±0.2 s.d. Green symbols show the ESCRT and related proteins that show fold change greater than ±0.2 s.d. (c) Western blot analysis of change in the cell membrane level of representative non-ESCRT proteins that were identified by MS analysis to be increased (Annexin A1- and Galectin-1) or not altered (Cadherin) at the cell surface by ionomycin-induced Ca2+increase. The molecular weight (KDa) markers are marked for each blot. (d) Plot showing average change in cell surface level of ESCRT proteins as assessed by MS analysis. Specific protein level were quantified by ion chromatogram of peptides (generated by IP2 Census quantitation software) such that the values for all peptides corresponding to a protein were averaged to obtain ratio shown for the abundance of this protein in Ionomycin versus DMSO treated cells—error bars represent s.d. (e) Representative western blots (n=3) with corresponding molecular weight (KDa) markers, and (f) averaged ratio for ionomycin triggered change in cell surface level of proteins in ESCRT III and accessory proteins—error bars represent s.e. Figure 1: Ca 2+ triggers recruitment of ESCRT III complex at the cell membrane. SILAC labelled and unlabelled C2C12 myoblasts treated for 5 min with Ionomycin (10 μM) or with DMSO (0.1%) were pooled, and the cell membrane proteins were extracted. ( a ) A representative coomassie-stained 1D SDS-PAGE gel ( n =6) used for differential cell membrane proteomic analysis. The gel shows molecular weight marker and the cell membrane protein pool (pooled lysate). The gel lane for pooled lysate was cut into slices and processed for proteomic analysis by mass spectrometry (MS). ( b ) Scatter (volcano) plot shows the fold change (log 2 average ratio) and –log 10 P value (one sample t -test versus ratio of 1.0) for the proteins quantified in at least two of the six independently replicated experiments. Black spots represent protein whose abundance was not altered in response to ionomycin-triggered Ca 2+ increase or the alteration did not reach the designated statistical significance across replicates. Red symbols represent proteins with P <0.06 (one sample t -test versus ratio of 1.0) and fold change ±0.4 s.d., whereas blue symbols mark proteins with P <0.06 and fold change ±0.2 s.d. Green symbols show the ESCRT and related proteins that show fold change greater than ±0.2 s.d. ( c ) Western blot analysis of change in the cell membrane level of representative non-ESCRT proteins that were identified by MS analysis to be increased (Annexin A1- and Galectin-1) or not altered (Cadherin) at the cell surface by ionomycin-induced Ca 2+ increase. The molecular weight (KDa) markers are marked for each blot. ( d ) Plot showing average change in cell surface level of ESCRT proteins as assessed by MS analysis. Specific protein level were quantified by ion chromatogram of peptides (generated by IP2 Census quantitation software) such that the values for all peptides corresponding to a protein were averaged to obtain ratio shown for the abundance of this protein in Ionomycin versus DMSO treated cells—error bars represent s.d. ( e ) Representative western blots ( n =3) with corresponding molecular weight (KDa) markers, and ( f ) averaged ratio for ionomycin triggered change in cell surface level of proteins in ESCRT III and accessory proteins—error bars represent s.e. Full size image The list of upregulated proteins identified by MS analysis included various endosomal proteins—notably ESCRT III members Chmp4B and Chmp1a were among the top 15 altered proteins ( Supplementary Data2 ). Chmp6 level also increased by 1.2-fold, but did not reach the applied statistical threshold of P value <0.06 ( Supplementary Data1 ). We also detected ESCRT-binding proteins—ALIX, Vps4 and ALG-2 ( Fig. 1b (green symbol), Fig. 1d ). However, we did not observe any proteins from traditional ESCRT 0, II and only member of the ESCRT I complex (Tsg-101). Therefore, we examined Ca 2+ -triggered changes in the cell surface level of all ESCRT complexes ESCRT 0 (STAM) ESCRT I (Vps37) and ESCRT II (Vps25) by WB. We found that Ca 2+ -triggered increase in cell surface level of ESCRT III and interacting proteins (including Tsg-101), but did not increase the cell membrane level of all proteins tested for ESCRT 0–II complexes ( Fig. 1e,f , Supplementary Fig. 1A ). To monitor the effect of ionomycin-induced global increase in cellular Ca 2+ level, we immunostained ESCRT proteins in untreated or ionomycin-treated cells. Ionomycin caused punctate distribution of both the ESCRT III-associated proteins tested (Vps4B and ALG-2), but it did not affect the distribution of ESCRT 0 member STAM, which remained diffusely distributed in the cytosol ( Supplementary Fig. 1B ). Next, we used live imaging to monitor the effect of Ca 2+ increase on localization of ESCRT III and associated proteins in myoblasts. Live total internal reflection fluorescenc (TIRF) imaging of cells showed that Chmp4B and Chmp1A puncate start forming at the cell surface within 90 s of being treated with ionomycin ( Supplementary Fig. 2A–D ). Similar response was observed for fluorescently tagged Vps4, Tsg101 and ALG-2 ( Supplementary Fig. 2E–L ). Together, the above observations show that Ca 2+ triggers rapid assembly of ESCRT III-Vps4 complex into punctae at the cell surface. Ca 2+ triggers ESCRT recruitment at the injured cell membrane Having established Ca 2+ -triggered cell surface accumulation of ESCRT III complex, we examined if injury triggered increase in Ca 2+ also leads to ESCRT accumulation at the cell membrane. Confocal or TIRF imaging of cell membrane following focal injury by a pulsed laser resulted in the accumulation of the punctae containing ESCRT III (Chmp1A and Chmp4B— Fig. 2a–d ) and accessory proteins ALG-2, ALIX and Vps4B ( Fig. 2e–j ) at the site of repair. This accumulation was dependent on the presence of extracellular calcium at the time of injury. Cells injured in the absence of extracellular Ca 2+ lacked any ESCRT accumulation or formation of any puncta. Moreover, owing to the lack of cell membrane repair, following injury these proteins also leaked from the cell resulting in injury-triggered decrease in their cellular level ( Fig. 2k–m ). In the presence of calcium, formation of the puncta initiated within the first minute and peaked over the next minute ( Fig. 2b,d,f,h,j ). Examination of the injury-triggered kinetics of puncta formation identified that punctae for ALG-2 and its binding partner ALIX began assembling within 30 s of injury, followed by Chmp (~45 s post injury) and Vps4B (~60 s) punctae ( Fig. 2n ). These differences in time of accumulation of ESCRT III and Vps4B were statistically significant as compared with ALG-2 and ALIX, but initiation of ALG-2 accumulation was indistinguishable from that of ALIX. 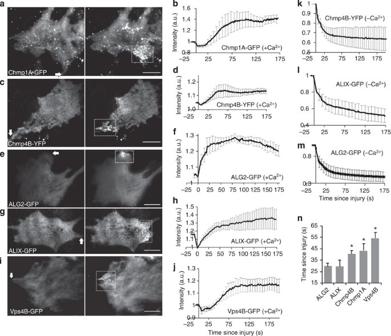Figure 2: Injury triggers recruitment of ESCRT III and accessory proteins at the site of repair. C2C12 myoblasts expressing fluorescently tagged (a,b) Chmp1A, (c,d) Chmp4B, (e,f) ALG-2, (g,h) ALIX and (i,j) Vps4B proteins were injured using a pulsed laser. Representative TIRF images (a,c,e,g,i) show change in the level of ESCRT and accessory proteins at the injured cell membrane. The kinetics of accumulation of these proteins at the injured cell membrane when cells were injured in the (b,d,f,h,j) presence or the (k,l,m) absence of extracellular calcium. Images show the cells 5 s before injury (pre-injury) and at the time point following injury when the intensity of the respective protein at the site of injury has reached its peak value (post-injury) and the plots show average ofn>4 cells each. (n) Kinetics of protein accumulation at the injured cell membrane was imaged and the chart shows average time each protein takes to initiate accumulation following injury (n>10 cells each). Arrows on the image show the site of injury and boxes mark the site of repair where proteins accumulate. Scale bars represent 10 μm and (*) representsPvalue <0.03 (paired two-tailedt-test with ALG-2) and error bars represent s.e. Figure 2: Injury triggers recruitment of ESCRT III and accessory proteins at the site of repair. C2C12 myoblasts expressing fluorescently tagged ( a , b ) Chmp1A, ( c , d ) Chmp4B, ( e , f ) ALG-2, ( g , h ) ALIX and ( i , j ) Vps4B proteins were injured using a pulsed laser. Representative TIRF images ( a , c , e , g , i ) show change in the level of ESCRT and accessory proteins at the injured cell membrane. The kinetics of accumulation of these proteins at the injured cell membrane when cells were injured in the ( b , d , f , h , j ) presence or the ( k , l , m ) absence of extracellular calcium. Images show the cells 5 s before injury (pre-injury) and at the time point following injury when the intensity of the respective protein at the site of injury has reached its peak value (post-injury) and the plots show average of n >4 cells each. ( n ) Kinetics of protein accumulation at the injured cell membrane was imaged and the chart shows average time each protein takes to initiate accumulation following injury ( n >10 cells each). Arrows on the image show the site of injury and boxes mark the site of repair where proteins accumulate. Scale bars represent 10 μm and (*) represents P value <0.03 (paired two-tailed t -test with ALG-2) and error bars represent s.e. Full size image ESCRT recruitment is independent of cell type and MVB To assess if ESCRT accumulation was unique to muscle cells, we assessed this in HeLa cells. For this we made use of HeLa cells stably expressing near endogenous levels of Chmp4B-GFP and Vps4A-GFP [24] . Both these and other proteins we assessed were found to accumulate at the site of repair in a manner similar to the myoblasts, indicating cell type independence of this response ( Fig. 3a,b ). 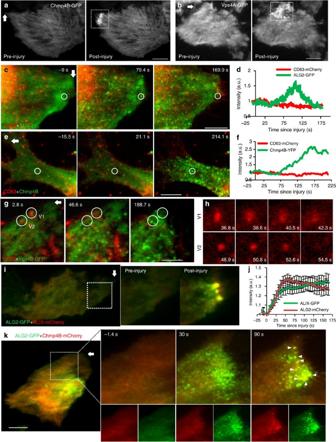Figure 3: ESCRT accumulation at injured cell membrane correlates with ALG-2 accumulation but not MVB fusion. HeLa cells stably expressing low levels of (a) Chmp4B-GFP and (b) Vps4A-GFP were injured by the pulsed laser at sites marked by the arrow. Images taken 5 s before injury (pre-injury) and at the peak of the respective protein accumulation (post-injury) show injury-triggered accumulation of these proteins similar to C2C12 cells. (c–f) HeLa cells co-expressing CD63-mCherry with (c,d) ALG2-GFP or (e,f) Chmp4B-YFP were injured by laser (marked by arrow) and accumulation of ALG2 and Chmp4B punctae (green) was monitored together with CD63 (red) by dual-color TIRF imaging. Plots show intensity of CD63 at the site of injury where individual ALG-2 or Chmp4B punctae (marked by white circles) form. Note that lack of colocalization between CD63-mCherry vesicle and the nascent ALG-2 or Chmp4B punctae. (g,h) Images of injury-triggered fusion of CD-mCherry (red) labelled vesicles (V1 and V2) together with accumulation of Vps4B-GFP (green) at the site of injury. Note that injury-triggered fusion of CD63-mCherry vesicles does not correlate spatially (V1) or temporally (V2) with formation of Vps4B puncate. (h) Images showing exocytosis of vesicles V1 and V2 as CD63-mCherry released by them diffuses into the cell membrane. (i) Images and (j) averaged plot (n=5) showing accumulation of ALG-2 mCherry and ALIX-GFP following focal laser injury. (k) Images showing accumulation of ALG-2 and Chmp4B in HeLa cell stably expressing Chmp4B-mCherry and transiently expressing ALG-2 following focal injury (white arrow). Zoom of the site of repair as ALG-2 (green) accumulates followed by Chmp4B (red) is shown and the individual channels (red and green) corresponding to the colour combined zoomed images are shown below each image. Scale bar represents 10 μm fora,b,iandk; 2 μm forc,eandg. Figure 3: ESCRT accumulation at injured cell membrane correlates with ALG-2 accumulation but not MVB fusion. HeLa cells stably expressing low levels of ( a ) Chmp4B-GFP and ( b ) Vps4A-GFP were injured by the pulsed laser at sites marked by the arrow. Images taken 5 s before injury (pre-injury) and at the peak of the respective protein accumulation (post-injury) show injury-triggered accumulation of these proteins similar to C2C12 cells. ( c – f ) HeLa cells co-expressing CD63-mCherry with ( c , d ) ALG2-GFP or ( e , f ) Chmp4B-YFP were injured by laser (marked by arrow) and accumulation of ALG2 and Chmp4B punctae (green) was monitored together with CD63 (red) by dual-color TIRF imaging. Plots show intensity of CD63 at the site of injury where individual ALG-2 or Chmp4B punctae (marked by white circles) form. Note that lack of colocalization between CD63-mCherry vesicle and the nascent ALG-2 or Chmp4B punctae. ( g , h ) Images of injury-triggered fusion of CD-mCherry (red) labelled vesicles (V1 and V2) together with accumulation of Vps4B-GFP (green) at the site of injury. Note that injury-triggered fusion of CD63-mCherry vesicles does not correlate spatially (V1) or temporally (V2) with formation of Vps4B puncate. ( h ) Images showing exocytosis of vesicles V1 and V2 as CD63-mCherry released by them diffuses into the cell membrane. ( i ) Images and ( j ) averaged plot ( n =5) showing accumulation of ALG-2 mCherry and ALIX-GFP following focal laser injury. ( k ) Images showing accumulation of ALG-2 and Chmp4B in HeLa cell stably expressing Chmp4B-mCherry and transiently expressing ALG-2 following focal injury (white arrow). Zoom of the site of repair as ALG-2 (green) accumulates followed by Chmp4B (red) is shown and the individual channels (red and green) corresponding to the colour combined zoomed images are shown below each image. Scale bar represents 10 μm for a , b , i and k ; 2 μm for c , e and g . Full size image We have previously shown that Ca 2+ triggers exocytosis of CD63-positive late endosomes [25] , [26] , a process associated with cell membrane repair [27] . Thus, although fusion of multivesicular body (MVB) leading to release of ILVs containing ESCRTs could provide a mechanism for the appearance of ESCRTs at the cell surface, the sequential nature of the assembly of ALIX, Chmp4B/Chpm1A and Vps4B ( Fig. 2n ) argues against such a possibility. To directly evaluate this possibility, we simultaneously imaged ESCRT appearance and fusion of CD63-mCherry-labelled MVBs. None of >30 nascent punctae, we monitored for each protein (ALG-2, Chmp4B or Vps4B), appeared coincident with CD63-labelled vesicles ( Fig. 3c–f ). Even when we monitored CD63-labelled vesicles that underwent injury-triggered exocytosis at the site of repair, the fusing vesicle did not deliver ESCRT puncta ( Fig. 3g,h ). These results show Ca 2+ -triggered MVB fusion is not the mechanism for ESCRT accumulation at the injured cell membrane. To directly examine if the sequential build-up of ESCRT III and accessory proteins involved their accumulation on the same location as ALG-2, we simultaneously expressed ALG-2 with low levels of ALIX or Chmp4B in the same cell. By monitoring injury-triggered accumulation of these proteins, we observed ALG-2-accumulated simultaneously (in space and time) with ALIX ( Fig. 3i,j ). However, this was different for the ESCRT III protein Chmp4B, which accumulated after ALG-2, but even here the nascent Chmp4B punctae colocalized with the ALG-2 punctae ( Fig. 3k ). This observation is reminiscent of sequential accumulation of ALIX and ESCRT III during other cellular processes regulated by ESCRTs [19] , [20] ( Supplementary Fig. 4 ). ALG-2 initiates ESCRT recruitment at injured cell membrane An important feature of ESCRT III accumulation at the injured cell membrane is its Ca 2+ -dependence. This could be on account of the EF-hand containing Ca 2+ -binding protein ALG-2 that has been shown to associate with ALIX, TSG-101 and Chmp4B in a Ca 2+ -dependent manner [28] . To examine if ALG-2 regulates Ca 2+ -triggered accumulation of ESCRTs, we tested if lack of ALG-2 affects injury-triggered accumulation of ESCRT III and accessory proteins. By use of ALG-2-targeted siRNA in HeLa cells, we reduced ALG-2 expression to well below 10% of the endogenous level ( Fig. 4a ). Unlike the control siRNA-transfected cells, the cells lacking ALG-2 expression failed to accumulate Vps4B ( Fig. 4b,c ) and Chmp4B ( Fig. 4d,e ) following injury. In view of the co-accumulation of ALG-2 with ALIX, we tested if ALG-2 regulates ALIX accumulation or if these two proteins accumulate independently. Again, whereas the control siRNA had no effect on ALIX accumulation, lack of ALG-2 prevented injury-triggered accumulation of ALIX ( Fig. 4f,g ). Although this indicates requirement of ALG-2 for ALIX accumulation, it is plausible that ALG-2 and ALIX may have complimentary role in their accumulation. In such an event, ALG-2 will have a regulatory function rather than a recruitment function, and each of these proteins will be needed for the co-accumulation. To test this possibility next, we generated a pool of HeLa cells stably expressing ALIX shRNA vector or the control empty shRNA vector. Cells with ALIX shRNA showed <10% of ALIX protein level as compared with the empty vector control cells ( Fig. 5a,b ). In view of the direct interaction between ALG-2 and ALIX, we tested the level of ALG-2 in the ALIX knocked down cells and found that ALIX knockdown does not affect the expression level of ALG-2 protein ( Fig. 5a,c ). We then assessed the effect of ALIX knockdown on injury-triggered ALG-2 accumulation and found that lack of ALIX did not prevent, but caused a slight delay in the accumulation of ALG-2 ( Fig. 5d,e ). Further, similar to the lack of ALG-2, lack of ALIX also prevented injury-triggered accumulation of Chmp4B ( Fig. 5f–g ) and Vps4B ( Fig. 5h,i ). Above observations that ALG-2 and ALIX are required for injury-triggered recruitment of ESCRT III and Vps4 complex, and following injury they begin accumulating before ESCRT III and Vps4 ( Fig. 2n ) point to sequential recruitment of injury-triggered ESCRT accumulation, which is initiated by ALG-2 and mediated by ALIX. 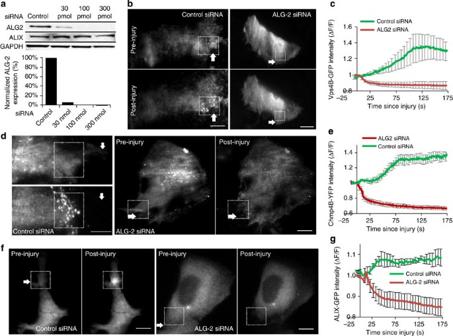Figure 4: ALG-2 is required for injury-triggered ALIX and ESCRT III assembly. Control and ALG-2 specific siRNAs were transfected in HeLa cells and its effect was assessed on (a) expression of ALG-2 and ALIX (seeSupplementary Fig. 5Afor uncropped blots), (b–g) injury-triggered accumulation of (b,c) Vps4B-GFP, (d,e) Chmp4B-YFP and (f,g) ALIX-GFP. TIRF images show cells 1 s before injury (pre-injury) and 125 s following injury (post-injury). Plots show change in intensity of indicated protein at the site of repair in four cells each. The site of injury is marked by white arrow, whereas the site of repair is marked by the dotted box. Scale bar represents 10 μm and the error bars indicate s.e. Figure 4: ALG-2 is required for injury-triggered ALIX and ESCRT III assembly. Control and ALG-2 specific siRNAs were transfected in HeLa cells and its effect was assessed on ( a ) expression of ALG-2 and ALIX (see Supplementary Fig. 5A for uncropped blots), ( b – g ) injury-triggered accumulation of ( b , c ) Vps4B-GFP, ( d , e ) Chmp4B-YFP and ( f , g ) ALIX-GFP. TIRF images show cells 1 s before injury (pre-injury) and 125 s following injury (post-injury). Plots show change in intensity of indicated protein at the site of repair in four cells each. The site of injury is marked by white arrow, whereas the site of repair is marked by the dotted box. Scale bar represents 10 μm and the error bars indicate s.e. 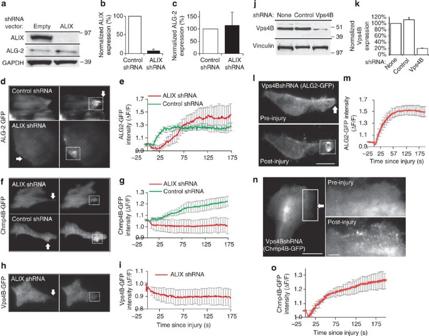Figure 5: ALIX regulates injury-triggered accumulation of ESCRT III but not of ALG-2. (a) Western blot analysis of ALIX and ALG-2 expression in HeLa cells stably expressing ALIX or empty shRNA vector (Supplementary Fig. 5Bshows uncropped blots). Quantification of averaged (b) ALIX, and (c) ALG-2 expression normalized to GAPDH from three independent experiments. (d–i) TIRF images and quantification of control and ALIX knockdown cells during the course of repair from laser injury (white arrow) to assess the effect on injury-triggered accumulation of (d,e) ALG2-GFP, (f,g) Chmp4B-GFP and (h,i) Vps4B-GFP at the site of repair. The plot shows the averaged values for change in the level of respective proteins within the site of repair contained by the dotted box. (j) Western blot analysis of Vps4B expression in HeLa cells stably expressing Vps4B shRNA or empty shRNA vector (Supplementary Fig. 5Bshows uncropped blots). (k) Quantification of averaged Vps4B expression normalized to GAPDH in three independent experiments. (i–o) TIRF images and quantification of injury-triggered accumulation of (l,m) ALG2-GFP, and (n,o) Chmp4B-GFP at the site of repair in Vps4B knockdown cells before and following repair from laser injury. Injury site is marked by white arrow and the plot shows the averaged values (n=5 cells) for the accumulation of respective proteins. Scale bar represents 10 μm and the error bars indicate s.e. Full size image Figure 5: ALIX regulates injury-triggered accumulation of ESCRT III but not of ALG-2. ( a ) Western blot analysis of ALIX and ALG-2 expression in HeLa cells stably expressing ALIX or empty shRNA vector ( Supplementary Fig. 5B shows uncropped blots). Quantification of averaged ( b ) ALIX, and ( c ) ALG-2 expression normalized to GAPDH from three independent experiments. ( d – i ) TIRF images and quantification of control and ALIX knockdown cells during the course of repair from laser injury (white arrow) to assess the effect on injury-triggered accumulation of ( d , e ) ALG2-GFP, ( f , g ) Chmp4B-GFP and ( h , i ) Vps4B-GFP at the site of repair. The plot shows the averaged values for change in the level of respective proteins within the site of repair contained by the dotted box. ( j ) Western blot analysis of Vps4B expression in HeLa cells stably expressing Vps4B shRNA or empty shRNA vector ( Supplementary Fig. 5B shows uncropped blots). ( k ) Quantification of averaged Vps4B expression normalized to GAPDH in three independent experiments. ( i – o ) TIRF images and quantification of injury-triggered accumulation of ( l , m ) ALG2-GFP, and ( n , o ) Chmp4B-GFP at the site of repair in Vps4B knockdown cells before and following repair from laser injury. Injury site is marked by white arrow and the plot shows the averaged values ( n =5 cells) for the accumulation of respective proteins. Scale bar represents 10 μm and the error bars indicate s.e. Full size image A key test of this model would be that preventing later events in the sequential recruitment pathway (ESCRT III/Vps4 recruitment) should not affect the earlier steps (ALG-2/ALIX recruitment). We thus examined the effect of the lack of Vps4B on Chmp4B and ALG-2 accumulation. For this, we generated a HeLa cell line stably knocked down for Vps4B to <10% of endogenous level ( Fig. 5j,k ). We observed that Vps4B depletion had no effect on injury-triggered accumulation of ALG-2 ( Fig. 5l,m ) or Chmp4B ( Fig. 5n,o ), indicating that Vps4B is dispensable for Chmp4B and ALG-2 accumulation. This finding thus establishes the sequential recruitment model for injury-triggered ESCRT III recruitment. ESCRTs facilitate repair of large cell membrane wound Although the ALG-2, ALIX and Vps4B knockdown each had different effects on injury-triggered recruitment of proteins, in all cases we observed increased number of cells failed to survive injury. This suggested that proper assembly of the entire ESCRT III-Vps4 complex is needed for proper repair of cell membrane to proceed. To examine this possibility, we assessed cell membrane repair using the commonly used assay of FM dye entry following laser injury [29] , [30] , which recapitulates the Ca 2+ -dependent repair of cell membrane injury [6] , [31] ( Supplementary Fig. 3A ). As a first step towards exploring the link between cell membrane repair and injury-triggered ESCRT assembly, we examined if cell membrane repair kinetics occurs at the same time scale as injury-triggered ESCRT III accumulation. Monitoring ESCRT III assembly using Chmp4B-GFP and repair by following entry of the FM4-64 dye, we observed Chmp4B accumulation at the site of repair coincides with that of cessation of FM dye entry, indicating efficient cell membrane repair ( Fig. 6a,b ). To examine if this correlation is causally linked with repair, we next assessed cell membrane repair in cells knocked down for the ESCRT III assembly and accessory proteins. 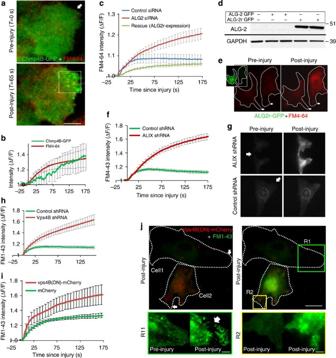Figure 6: Ca2+-triggered ESCRT/Vps4B assembly allows cell membrane repair. Following laser injury of myoblasts in the presence of FM dye, repair of cell membrane was monitored by following dye entry, which results in increase in FM-dye fluorescence. Cellular dye fluorescence was normalized to the time point before injury (ΔF/F). (a) Live cell TIRF (green) and widefield (red) images of a myoblast expressing Chmp4B-GFP (green) and injured in the presence of FM4-64 dye (red) by laser (arrow). (b) The plot shows kinetics of cell membrane repair (FM 4–64 intensity) and Chm4B-GFP accumulation at the injured cell membrane. (c) Plot showing FM 4–64 entry following laser injury of 10–12 cells transfected for 72 h with control siRNA (blue line), ALG-2 siRNA with no subsequent treatment (red line), or subsequent transfection with siRNA resistant ALG2-GFP plasmid (ALG2r-GFP). (d) Western blot analysis of expression of ALG2-GFP and ALG2r-GFP in cell lysates from HeLa cells transfected with these plasmids with or without ALG-2 siRNA and probed with ALG2 antibody. Bands corresponding to the GFP-tagged protein are shown here and the uncropped blots are shown inSupplementary Fig. 5C(e) Images showing laser injury-induced uptake of FM4-64 dye (red) in HeLa cells expressing or not expressing ALG2r-GFP (inset, green cell). (f) Kinetics of injury-triggered FM 1–43 entry in stable clones of HeLa cells expressing ALIX shRNA (red symbol) or empty vector (control; green symbol) averaged for 10–15 cells in each condition. (g) Representative images of a pair of ALIX shRNA or empty vector control cells injured (at the site marked by the arrow) in the presence of FM 1–43 dye. (h) Kinetics of injury-triggered FM 1–43 entry in stable clones of HeLa cells expressing Vps4B shRNA (red symbol) or empty vector (control; green symbol) averaged for 10–15 cells in each condition. (i) Kinetics of injury-triggered FM 1–43 entry in up to 15 C2C12 myoblasts each transiently expressing mCherry (green) or Vps4B(DN)-mCherry. (j) Representative images of FM1-43 dye entry following injury of a pair of C2C12 myoblasts expressing (Cell2) or not expressing (Cell1) Vps4B(DN)-mCherry for 24 h. Zoomed inset R1 and R2 show the region near the site of injury for cell 1 (lacking) and cell 2 (expressing) Vps4B(DN)-mCherry. Arrow in R1 shows the site where the damaged membrane was excised from the repaired cell and the diffraction limited dots represent the vesicles released during excision of the membrane. Error bars represent s.e., and scale bars represent 10 μm for the whole-cell images and 2 μm for the zoomed regions R1 and R2. Figure 6: Ca2+-triggered ESCRT/Vps4B assembly allows cell membrane repair. Following laser injury of myoblasts in the presence of FM dye, repair of cell membrane was monitored by following dye entry, which results in increase in FM-dye fluorescence. Cellular dye fluorescence was normalized to the time point before injury (ΔF/F). ( a ) Live cell TIRF (green) and widefield (red) images of a myoblast expressing Chmp4B-GFP (green) and injured in the presence of FM4-64 dye (red) by laser (arrow). ( b ) The plot shows kinetics of cell membrane repair (FM 4–64 intensity) and Chm4B-GFP accumulation at the injured cell membrane. ( c ) Plot showing FM 4–64 entry following laser injury of 10–12 cells transfected for 72 h with control siRNA (blue line), ALG-2 siRNA with no subsequent treatment (red line), or subsequent transfection with siRNA resistant ALG2-GFP plasmid (ALG2r-GFP). ( d ) Western blot analysis of expression of ALG2-GFP and ALG2r-GFP in cell lysates from HeLa cells transfected with these plasmids with or without ALG-2 siRNA and probed with ALG2 antibody. Bands corresponding to the GFP-tagged protein are shown here and the uncropped blots are shown in Supplementary Fig. 5C ( e ) Images showing laser injury-induced uptake of FM4-64 dye (red) in HeLa cells expressing or not expressing ALG2r-GFP (inset, green cell). ( f ) Kinetics of injury-triggered FM 1–43 entry in stable clones of HeLa cells expressing ALIX shRNA (red symbol) or empty vector (control; green symbol) averaged for 10–15 cells in each condition. ( g ) Representative images of a pair of ALIX shRNA or empty vector control cells injured (at the site marked by the arrow) in the presence of FM 1–43 dye. ( h ) Kinetics of injury-triggered FM 1–43 entry in stable clones of HeLa cells expressing Vps4B shRNA (red symbol) or empty vector (control; green symbol) averaged for 10–15 cells in each condition. ( i ) Kinetics of injury-triggered FM 1–43 entry in up to 15 C2C12 myoblasts each transiently expressing mCherry (green) or Vps4B(DN)-mCherry. ( j ) Representative images of FM1-43 dye entry following injury of a pair of C2C12 myoblasts expressing (Cell2) or not expressing (Cell1) Vps4B(DN)-mCherry for 24 h. Zoomed inset R1 and R2 show the region near the site of injury for cell 1 (lacking) and cell 2 (expressing) Vps4B(DN)-mCherry. Arrow in R1 shows the site where the damaged membrane was excised from the repaired cell and the diffraction limited dots represent the vesicles released during excision of the membrane. Error bars represent s.e., and scale bars represent 10 μm for the whole-cell images and 2 μm for the zoomed regions R1 and R2. Full size image In view of the role of ALG-2 in initiating injury-triggered ESCRT assembly, we first examined the effect of ALG-2 knockdown. Whereas control siRNA expressing cells repaired within a minute of injury, cells depleted for ALG-2 failed to prevent FM-dye entry ( Fig. 6c , red plot; Supplementary Fig. 3B ). To assess the specificity of the response, we generated ALG-2 cDNA (ALG-2r) that is unaffected by the ALG-2 siRNA used in this study ( Fig. 6d ). Expression of GFP-tagged ALG-2r (ALG2r-GFP) rescued the repair defect caused by siRNA-mediated knockdown of ALG-2 ( Fig. 6e , c-green plot). This establishes a need of ALG-2 in repair of injured cell membrane. We next assessed the role of ALIX in this process. Similar to ALG-2, cells lacking ALIX failed to repair from a focal laser injury ( Fig. 6f,g ). These results indicate that independent of the approach used, blocking injury-triggered ESCRT assembly prevents repair of the injured cells. We next tested if ESCRT III assembly alone is sufficient for repair or repair also requires assembly of the Vps4 complex. To address this, we used two complimentary approaches. In the first approach, we used HeLa cells knocked down for Vps4B and found that cells lacking Vps4B failed to repair from injury ( Fig. 6h ). In the second approach, we monitored repair of HeLa cells by blocking Vps4 function by the expression of dominant negative Vps4B cDNA—Vps4B(DN) mutant [32] . Compared with cells expressing mCherry protein ( Fig. 6i ) or no exogenous proteins ( Fig. 6j ) cells that expressed Vps4B(DN)-mCherry for as little as 16 h failed to repair and prevent FM dye entry ( Fig. 6i,j ). The need for Vps4B activity is suggested by a closer comparison of the fate of the cell membrane at the site of injury (R1, R2). Whereas R1 (not expressing Vps4B(DN)) shows the injured part of the cell membrane was excised from the rest of the repaired cell and fragmented into smaller vesicles ( Fig. 6j zoom of post-repair R1 image), in the case of R2 (the cell expressing Vps4B(DN)), the injured part of the membrane remained contiguous with the rest of the cell body and no vesicles were shed by the injured cell membrane. This latter behaviour is similar to what we observed for cells injured in the absence of calcium ( Supplementary Fig. 3A , R1 versus R2) as well as cells lacking ALG2 or Vps4B expression ( Supplementary Fig. 3B ,C—region R3 versus R4 and R5 versus R6). In view of the known role of ESCRT III-Vps4B complex in membrane scission above observation indicate that membrane scission and vesiculation is required for repair and is mediated by ESCRT III-Vps4B complex. We next examined if shedding of the vesicles also occurs following injury of muscle fibres in an intact muscle tissue. For this, we used intact biceps muscle and carried out focal ex vivo injury of individual myofibres in the intact muscle using pulsed laser in the presence of FM1-43 dye to label the cell membrane and all of the released extracellular vesicles. Following injury, we observed as the injured myofibres repaired they shed FM dye-labelled vesicles into the endomysial space and these vesicles originated from the site of injury ( Supplementary Movie 1 , Supplementary Fig. 3D,E ). As with the ESCRT III assembly ( Fig. 6a,b ), we found that the time course of extracellular vesicle shedding by the injured myofibre (indicated by red line in Supplementary Fig. 3E ) occurred co-incident with the repair of the damaged cell membrane—as indicated by plateauing of FM dye entry in the cell ( Supplementary Fig. 3E ). This indicates that the Ca 2+ -triggered vesiculation to remove damaged membrane is a phenomenon that extends beyond the mononucleate muscle cells not only to other types of mononucleated cells, but also multinucleate muscle fibres that have fully differentiated in vivo . ESCRT complex is involved in cell membrane repair in a manner that closely parallels the involvement of this complex in retroviral budding and cytokinesis ( Supplementary Fig. 4 ). Similar to these latter processes, injury triggers sequential assembly of ESCRT III without triggering assembly of most of the known ESCRTs 0-II member. ESCRT assembly at the injured cell membrane is dependent on ALIX ( Fig. 5a–c ). It is suggested that following injury ALIX may associate with cell membrane through its endosomal lipid (LBPA—lysobisphosphatidic acid)-binding domain [11] . However, we find that injury-triggered ALIX accumulation depends on ALG-2, absence of which prevents ALIX accumulation ( Fig. 4f,g ). As accumulation of ALG-2 itself is not prevented by the lack of ALIX ( Fig. 5d,e ), ALG-2 appears to be the regulator of ALIX accumulation and not vice versa. However, both ALG-2 and ALIX are needed for the accumulation of ESCRT III and Vps4 complexes at the injured cell membrane ( Figs 4 and 5 ). On the basis of these features, we conclude that ALG-2 is the initiator and its binding partner ALIX is the facilitator of ESCRT III recruitment. Binding between ALIX and ALG-2 occurs through a motif in ALIX that partially overlaps with that of Cep55 (centrosome protein of 55 kDa)—the protein responsible for ESCRT III assembly during cytokinesis [33] . By the virtue of its ability to form a homodimer, ALG-2 can function as an adaptor bridging two interacting proteins such as ALIX and Tsg101 (ref. 34 ). This could be the basis for the presence of Tsg101—the sole ESCRT I/ESCRT II protein to accumulate at the site of cell membrane repair. In view of above, the role of ALG-2 during cell membrane repair appears to parallel that of Cep55 during cytokinesis and Gag during HIV budding. As these are ESCRT 0 proteins (for their respective processes), we propose that ALG-2 is the ESCRT 0 protein for cell membrane repair ( Supplementary Fig. 4 ). ALG-2 is among the best conserved penta-EF hand protein. Penta-EF domain contains an evolutionarily primitive Ca 2+ -binding motif found in a number of protein families including calpains and S100 proteins. Calpain has been implicated in the repair of injured cell membrane [35] and we have recently identified a similar role for S100 protein—S100A11 (ref. 36 ). Identification of a role of ALG-2 in cell membrane repair adds further to the importance of EF hand proteins in facilitating cell membrane repair. As cell membrane injury is arguably among the earliest and ubiquitous calcium-dependent cellular process, the ancient origin and widespread presence of EF hand in proteins may have facilitated their use to sense injury-triggered calcium entry and initiate a repair response. So far, the only function attributed to the calcium-binding ability of ALG-2 has been the Ca 2+ sensor at ER exit sites, where it stabilizes membrane association of Sec31 and facilitates ER exit [37] . Our finding that ALG-2 can assemble at injured cell membrane in response to Ca 2+ increase identifies a new feature of this protein, which we find is needed for repair of injured cell membrane. Further, ALG-2 involvement in repair is noteworthy owing to the initial identification of ALG-2 as a Ca 2+ -dependent regulator of cell death [16] . Although cells that fail to repair will undergo necrotic cell death, we believe that ALG-2 may regulate the activation of cell death in those cell that close the cell membrane breach, but fail to fully recover from the injury. Such a role of ALG-2 will be of great relevance to disease models where cell membrane repair is inefficient [6] , [38] . ALG-2 and ALIX mediated ESCRT III and Vps4 accumulation facilitates cleavage of injured cell membrane. Cell membrane cleavage proceeds with the involvement of ESCRT III and Vps4 complex. Accumulation of Vps4 is required for the cleavage of damaged region of the injured cell membrane, as lack of Vps4 and blocking its function by use of dominant negative Vps4 prevents cleavage of the injured cell membrane ( Fig. 6h–j and Supplementary Fig. S3B,C ). Cleavage of injured cell membrane results in the formation of small extracellular vesicles that are shed from the site of injury in cultured cells and in muscle tissue ( Fig. 6j , Supplementary Fig. 3 ). Shedding of injured cell membrane as small extracellular vesicles by ESCRT III-Vps4 complex is distinct from blebbing of injured cell membrane and from our recent demonstration of actin-mediated large-scale retraction of damaged cell membrane [36] , [39] . Formation and shedding of extracellular vesicles is a key step in the process of regulating tissue inflammation and repair following injury [40] . Thus, in addition to facilitating repair of the injured cell membrane, involvement of ESCRT-mediated shedding of injured cell membrane may also aid tissue repair by activating inflammatory signalling through the release of extracellular vesicles. In summary, results presented here point to the role of ESCRTs in repair of large focal injuries and identify the sequential process by which ESCRT III and Vps4 complexes are assembled at the site of injury. It remains to be seen if this mechanism is conserved even in case of small cell membrane injuries such as by the pore-forming toxins. In addition, work using knockout mouse models would help address the in vivo role of ESCRTs in the repair and regeneration of muscles injured by exercise or due to genetic deficits. With increasing recognition of extracellular vesicles in the process of tissue inflammation and repair, ESCRT-mediated vesiculation could also offer insights into extracellular signalling required to initiate inflammation and stem cell activation for efficient regeneration of muscle and other tissues. Cell culture Mouse C2C12 myoblasts (ATCC, Manassas, VA, USA) were routinely cultured in Dulbecco’s modified eagle medium (DMEM) with Glutamax, high glucose, 110 mg l –1 sodium pyruvate (Invitrogen, Carlsbad, CA, USA) supplemented with 10% fetal bovine serum (Hyclone, Thermo Fisher Scientific, USA) and with 100 μg ml –1 Penicillin and 100 μg ml –1 Streptomycin (Invitrogen) at 37 °C and 5% CO 2 . HeLa cells (ATCC) and clones stably expressing low levels of specific ESCRT proteins [24] were grown in DMEM (without pyruvate, Gibco, catalog number 11965-092) with 10% fetal bovine serum and 0.4 μg ml –1 Geneticin at 37 °C and 5% CO 2 using standard sterile techniques. For SILAC, labelling cells were cultured for six generations in media containing regular Lysine and Arginine isotopes (unlabelled) or with media that has 13 C 6 arginine and 15 N 2 , 13 C 6 Lysine as the sole source of these amino acids (labelled). To test complete replacement of lysines and arginine by their heavy counterparts, C2C12 cells were cultured in the presence of 13 C 6 arginine and 15 N 2 , 13 C 6 Lysine as described above and all proteins from five random gel slices from five different locations of the gel for a crude protein extract were subjected to tryptic digestion. The resulting peptide mixture was analyzed by MS, which showed a >99% incorporation of the SILAC label. These labelled cells were then used for subsequent treatment and preparation of plasma membrane proteome along with unlabelled cells cultured simultaneously in unlabelled media. Plasmids and stable cell lines C2C12 or Hela were transfected with the indicated plasmid using Lipofectamine LTX (Life technologies) or Fugene 6 (Roche Biochemicals), respectively, as per manufacterers’ instructions. Expression was allowed for 24–48 h. The plasmids used to make stably expressing/knocked down HeLa cell lines are based on the pLNCX2 plasmid (Clontech) with GFP-Chmp4B, GFP-Vps4A (A gift by Sanford Simon [24] ) or shRNA-Vps4B (A gift from Yasuo Ariumi). The open reading frame was sequenced completely. The following retroviral constructs were used for this study: pLNCX2-mEGFP-Chmp4B (NM_176812), pLNCX2-mEGFP-Vps4A [19] , pLV-Vps4Bi, pLV-ALIXi and non-targeting control shRNA sequence pLV-shCon as described elsewhere [41] . Sense and antisense sequences of the oligonucleotides used for the Vps4B shRNA and the production and use of the lentiviruses as described previously [41] and in Table 1 . Stable HeLa cell lines expressing tagged ESCRTs or vps4A shRNA were created and tested for any detectable adverse effects on cell growth. Retroviral vectors expressing the desired shRNA were transfected into HEK293T cells with plasmids expressing VSVG and MLV-Gag-Pol using Fugene 6 according to manufacturers’ instructions. Viruses were collected 24 h later, filtered through a 0.45-μm Millex HP PES filter (Millipore) and added to HeLa cells. 24 h later, selection was started using 400 μg ml –1 Geneticin (Invitrogen) and continued for at least 1 week. Clones expressing low levels of the protein or knocked down for vps4B were selected by limiting dilution. The clones selected also showed no morphological aberration and obvious difference in growth. ALG-2 siRNA used has been described in Table 1 . Table 1 shRNAs and siRNAs used in the study. Full size table To generate siRNA resistant ALG2, the cDNA was mutated to create four conservative point mutations (indicated in lowercase): 5′-GaUCcAUaAUcUCCAUGUU-3′. Once the ability of the mutated ALG-2 cDNA to avoid siRNA silencing was established at the protein level, this plasmid was used for functional rescue experiments for endogenous ALG-2. The siRNA was custom synthesized by Dharmacon (Thermo Scientific, USA). For control siRNA, siGLO RISC-free control siRNA (Thermo Scientific) were used. Hela cells were transfected with 300 pmol of siRNAs using oligofectamine according to manufacturers’ instructions. Ionomycin treatment and SILAC labelling To label cells using the SILAC strategy, DMEM media without lysine and arginine was custom prepared (Atlanta Biologicals, Lawrenceville, GA, USA), and complete unlabelled and labelled media was then constituted by the addition of either unlabelled lysine and arginine or 13 C 6 arginine (147.5 mg ml –1 ) and 15 N 2 , 13 C 6 Lysine (91.25 mg ml –1 ) (Cambridge Isotope Laboratories Inc., Andover, MA, USA), respectively, along with 10% fetal bovine serum (Hyclone, Thermo Fisher Scientific) and 100 mg ml –1 each of penicillin and streptomycin (Invitrogen), to the above lysine, arginine-depleted medium. Equal number of C2C12 cells grown in parallel in both labelled and unlabelled media for more than six passages to ensure labelling of all cellular proteins. Subsequently, the cell surface proteins present in both labelled and unlabelled cells were biotinylated using the protocol previously described [4] , following which labelled/unlabelled cells were treated at room temperature for 5 min with 15 ml Hank’s Balanced Salt solution (HBSS) containing 10 μM ionomycin, whereas corresponding unlabelled/labelled cells were treated at room temperature for 5 min with 15 ml of HBSS containing 0.1% DMSO. Of the six independent experiments in five experiments, labelled cells were treated with ionomycin and the unlabelled cells were treated with DMSO and this was reversed for one experimental replicate. Plasma membrane protein enrichment Plasma membrane proteins were purified from C2C12 myoblasts as previously described [4] . In brief, the cells were washed once with HBSS, scraped and unlabelled and labelled cells were mixed in a ratio of 1:1. Cells were then collected by ultracentrifugation (>200,000 g , 20 min, 4 °C) and the pellet was resuspended in 2 ml of HBSS. The cell suspension was homogenized in a tight-fitting 7 ml Dounce homogenizer with 20 strokes of pestle A and 50 strokes of pestle B. The homogenate was then centrifuged at 800 g , for 10 min at 4 °C to obtain the post-nuclear supernatant. The protein concentration was estimated in this supernatant using the Bio-Rad DC protein assay kit (Bio-Rad, Hercules, CA, USA). Subsequently, supernatant containing 1.3–2 mg protein was bound to streptavidin beads. The beads were then successively washed with a high salt and a high pH buffer, and finally rinsed twice with water. The beads were resuspended in 2 × sodium dodecyl sulfate sample buffer containing 2.5% β-mercaptoethanol. Sample preparation, in-gel digestion and peptide extraction The streptavidin beads containing bound biotinylated cell surface proteins were heated at 50 °C for 30 min to elute the proteins bound to the beads and 1D protein separation was performed using a precast 4–12% sodium dodecyl sulfate polyacrylamide gel electrophoresis gel (b is - tris Novex mini gel, Invitrogen). The gel was fixed with methanol:water:acetic acid (45:50:5 v/v/v) and subsequently bands were visualized by staining with coomassie blue (Bio-Rad). The fractionated gel lane was excised into 35 bands. Each slice was destained with 50% acetonitrile (ACN) (v/v) and 100 mM NH 4 HCO 3 , dehydrated with 100% ACN. Gel pieces were rehydrated in 10–20 μl of cold digestion buffer (12.5 ng μl –1 of gold-grade trypsin (Promega, Madison, WI, USA) in 50 mM NH 4 HCO 3 ) and incubated at 4 °C for 45 min. The excess buffer was removed and replaced with 50 mM NH 4 HCO 3 . Digestion with trypsin was carried out overnight at 37 °C. Tryptic peptides were extracted with 50% ACN with 5% formic acid, repeated twice. Pooled peptides were dried by vacuum centrifugation and resuspended in 10 μl of 0.1% trifluoroacetic acid. LC-MS/MS All analyses were carried out on a hybrid Thermo LTQ-OrbitrapXL (San Jose, CA, USA) mass spectrometer coupled online to an Eksigent nano-LC system (AB Sciex, Framingham, MA, USA). Each sample was injected via an autosampler and loaded onto a Symmetry C18 trap column (5 μm, 300 μm i.d. × 23 mm, Waters, Milford, MA, USA) for 10 min at a flow rate of 10 μl min –1 in high-performance liquid chromatography grade water with 0.1% formic acid. The sample was subsequently separated by a C18 reverse-phase column (3 μm, 200A, 100 μm × 15 cm, Magic C18, Michrom Bioresources) at a flow rate of 300 nl min –1 . The mobile phases consisted of water with 0.1% formic acid (A) and 90% ACN (B). A 65 min linear gradient from 5 to 40% B was used. Eluted peptides were introduced into the mass spectrometer via Michrom Bioresources CaptiveSpray (Bruker, Freemont, CA, USA). The spray voltage was set at 1.4 kV and the heated capillary at 200 °C. The LTQ-Orbitrap-XL was operated in data-dependent mode with dynamic exclusion in which one cycle of experiments consisted of a full-MS in the Orbitrap (300–2,000 m z –1 ) survey scan in profile mode, resolution 30,000, and five subsequent MS/MS scans in the LTQ of the most intense peaks in centroid mode using collision-induced dissociation with the collision gas (helium) and normalized collision energy value set at 35%. Database search and IP2 analysis For protein identification and quantification, we used Integrated Proteomics Pipeline (IP2) version 1.01 software developed by Integrated Proteomics Applications, Inc. ( http://www.integratedproteomics.com/ ). Mass spectral data were uploaded into IP2 software. Files from each lane were searched against the forward and reverse Uniprot mouse database (UniProt release 2010_12 with 16,333 entries) for partially tryptic peptides allowing one missed cleavage, and possible modification of oxidized methionine (15.99492 Da), heavy arginine (6.0204 Da) and heavy lysine (8.0142 Da). IP2 uses the Sequest 2010 (06_10_13_1836) search engine. Mass tolerances were set at ±30 ppm for MS and ±1.5 Da for MS/MS. Data were filtered on the basis of a 1% protein-false discovery rate. All the bands from each lane were summed in the analysis. Census software version 1.77, built into the IP2 platform, was used to determine the ratios of unlabelled and labelled peptide pairs using an extracted chromatogram approach. The distribution of ratios was plotted and correction factors applied to adjust for error in sample mixing. Data were checked for validity by using regression correlation better than 0.5 for each peptide pair. Bioinformatics analysis Biological replicates were combined in IP2 software using Quantitation Compare, which calculates the average ratio along with relative standard deviation and t -test P values. Proteins and corresponding quantitative ratios were filtered on the basis of identification and quantitation in at least two replicates, ratio ≥1.15 or ≤0.87 and t -test P value <0.059. Protein annotations were acquired using the Keyword and GO terms in the Uniprot Protein Knowledgebase ( http://www.uniprot.org/ ). Proteins of interest were further validated using alternative approaches. Immunoblot and immunostaining Cells were lysed with RIPA (Sigma Aldrich, St Louis, MO, USA) containing protease inhibitor cocktail (Fisher Scientific) for WB analysis or fixed with 4% paraformaldehyde or chilled methanol for immunofluorescence analysis. For WB, proteins were transferred to nitrocellulose membranes and probed with indicated primary antibody: Chmp4B (ab105768-1:1,000 dilution, Abcam, Cambridge, MA, USA); STAM (ab76061, 1:300, Abcam); Vps4B (SAB4200023, 1:500 dilution, Sigma Aldrich); Chmp1A (15761-1-AP, 1:500 dilution, Proteintech, Chicago, IL, USA); and Vps25 (15669-1-AP, 1:500 dilution, Proteintech), ALG-2 (H00010016-M01, 1:500 dilution, Novus Biologicals, Littleton, CO, USA) and Vps37C (NBP1-56409, 1:500 dilution, Novus Biologicals), Galectin-1 (AF1245, 1:500 dilution, R&D systems, Minneapolis, MN, USA), Cadherin (4068, 1/1,000 dilution, Cell Signaling Technology, Danvers, MA, USA), ALIX (sc-49268, 1:500 dilution, Santa Cruz Biotech, Dallas, TX, USA), Tsg-101 (sc-7964, 1:500 dilution, Santa Cruz Biotech). This was followed by probing with horseradish peroxidase-conjugated secondary antibodies (Sigma Aldrich), chemiluminescent western blotting substrate (Fisher, GE Healthcare, USA) and processed on Bio-Lite X-ray film and scanned and quantified by densitometry using BioRad GS-800 densitometer and normalized to the loading control to obtain ionomycin/DMSO fold change values. Uncropped blots corresponding to Figs 4 , 5 , 6 are shown in Supplementary Fig. 5 . For immunostaining, permeabilized cells were bound with appropriate antibodies followed by fluorophore-conjugated secondary antibodies: Alexa Fluor 488 anti-rabbit, Alexa Fluor 594 anti-rat and Alexa Fluor 594 anti-mouse (Life technologies). Nuclei were counterstained with Hoechst 33342. After mounting in the mounting medium (Dako, USA), cells were imaged with appropriate filters and × 60-1.45 numerical aperture objective on Olympus IX81 widefield microscope equipped with Orca-R2 camera (Hamamatsu Photonics, Japan). Live imaging For laser injury assay, cells cultured on coverslips were transferred in cell imaging media (CIM; HBSS with 10 mM HEPES pH 7.4) or phosphate-buffered saline (Sigma Aldrich) into Tokai Hit microscopy stage top ZILCS incubator (Tokai Hit Co., Japan) maintained at 37 °C. For laser injury, a 1–2 μm 2 area was irradiated for <100 ms with a pulsed laser (Ablate!, 3i Intelligent Imaging Innovations, Inc. Denver, CO, USA). To monitor ESCRT kinetics, cells expressing appropriate tagged ESCRT protein was injured and imaged in spinning disc confocal or TIRF mode using IX81 Olympus microscope (Olympus America, PA, USA) equipped with Yokogawa spinning disc confocal or Cell-TIRF (Olympus, PA, USA) system, respectively. For all, imaging a 60X-1.45 numerical aperture oil objective was used. To quantify cell membrane repair, 1 ug μl –1 FM1-43 dye (Life technologies) was added to the cell-imaging buffer used and cells were imaged at 10 s intervals using IX81 Olympus microscope (Olympus). FM dye intensity was used to quantify the kinetics of cell membrane repair. Mouse muscle isolation and membrane injury: methods involving animals were approved by the local institutional animal research committee, and animals were maintained in a facility accredited by the American Association for Accreditation of Laboratory Animal Care. Biceps muscle were surgically isolated from euthanized 3-month-old C57BL/6 mice in Tyrode’s solution containing 128 mM NaCl, 4.7 mM KCl, 1.36 mM CaCl2, 20 mM NaHCO3, 0.36 mM NaH2PO4, 1 mM MgCl2 and 10 mM glucose (pH 7.4). Laser injury was carried out as described above in the Tyrode’s buffer containing 1.33 μg μl –1 FM1-43 dye. How to cite this article: Scheffer, L. L. et al. Mechanism of Ca 2+ -triggered ESCRT assembly and regulation of cell membrane repair. Nat. Commun. 5:5646 doi: 10.1038/ncomms6646 (2014).